High oxide-ion conductivity through the interstitial oxygen site in Ba7Nb4MoO20-based hexagonal perovskite related oxides Oxide-ion conductors are important in various applications such as solid-oxide fuel cells. Although zirconia-based materials are widely utilized, there remains a strong motivation to discover electrolyte materials with higher conductivity that lowers the working temperature of fuel cells, reducing cost. Oxide-ion conductors with hexagonal perovskite related structures are rare. Herein, we report oxide-ion conductors based on a hexagonal perovskite-related oxide Ba 7 Nb 4 MoO 20 . Ba 7 Nb 3.9 Mo 1.1 O 20.05 shows a wide stability range and predominantly oxide-ion conduction in an oxygen partial pressure range from 2 × 10 −26 to 1 atm at 600 °C. Surprisingly, bulk conductivity of Ba 7 Nb 3.9 Mo 1.1 O 20.05 , 5.8 × 10 −4 S cm −1 , is remarkably high at 310 °C, and higher than Bi 2 O 3 - and zirconia-based materials. The high conductivity of Ba 7 Nb 3.9 Mo 1.1 O 20.05 is attributable to the interstitial-O5 oxygen site, providing two-dimensional oxide-ion O1−O5 interstitialcy diffusion through lattice-O1 and interstitial-O5 sites in the oxygen-deficient layer, and low activation energy for oxide-ion conductivity. Present findings demonstrate the ability of hexagonal perovskite related oxides as superior oxide-ion conductors. Oxide-ion conducting ceramic materials have attracted much attention due to their applications in solid-oxide fuel cells (SOFCs), oxygen separation membranes, gas sensors, and catalysts [1] , [2] , [3] , [4] , [5] , [6] , [7] , [8] , [9] , [10] , [11] , [12] , [13] , [14] , [15] , [16] , [17] , [18] , [19] , [20] , [21] , [22] , [23] , [24] . Yttria stabilized zirconia (YSZ) ceramics have widely been used, but the working temperature is high (700–1000 °C). Thus, there remains a strong motivation to explore oxide-ion conductors with higher conductivities at temperatures below 600 °C. High oxide-ion conductivities have been observed in specific structure families such as the fluorite-type, perovskite-type, melilite-type, and apatite-type structures [1] , [2] , [3] , [4] , [5] , [6] , [7] , [8] , [9] , [10] , [11] , [12] , [13] , [14] , [15] , [16] , [17] , [18] , [19] , [20] , [21] , [22] , [23] , [24] . The perovskite and its related materials exhibit interesting physical and chemical properties [25] and can be classified into four structural groups of (i) AMX 3 perovskite-type, (ii) AMX 3 -related, (iii) hexagonal perovskite-related and (iv) modular structures [26] where A and M are larger and smaller cations, respectively, and X is an anion. A number of perovskite-type materials and perovskite related phases belonging to the groups of (i), (ii) and (iv) have been reported to be oxide-ion conductors. The hexagonal perovskite-related structures (iii) have hexagonal close packing of AX 3 layers or sequences of hexagonal (h) and cubic (c) AX 3 (and/or anion-deficient AX 3– x (c′) where x is the anion vacancy content) close-packed layers. The hexagonal perovskite related oxides exhibit a variety of crystal structures [26] , [27] , [28] , [29] , [30] , [31] . However, oxide-ion conductors with hexagonal perovskite-related structures are quite rare. Several mixed ion (oxide-ion and/or proton) and electronic conductors with hexagonal perovskite related structures were reported in the literature [32] , [33] , [34] , [35] . The hexagonal perovskite related oxides Ba 3 M NbO 8.5– δ ( M = Mo and W; δ is the oxygen deficiency) and their solid solutions exhibit significant oxide-ion conductivities [23] , [30] , [31] , [36] , [37] , [38] , [39] , however, the conductivities are not high at temperatures below 600 °C. The relatively low conductivities are ascribed to relatively high activation energy for conductivity (e.g., 1.2 eV for Ba 3 MoNbO 8.5– δ [23] ). Therefore, we have explored oxide-ion conductors with the hexagonal perovskite related structures. Ba 7 Nb 4 MoO 20 is a trigonal \(P\bar 3m1\) hexagonal perovskite polytype 7H [29] , [40] . Fop et al. found high oxide-ion and proton conductivities of Ba 7 Nb 4 MoO 20 [40] . Herein, we report higher oxide-ion conductivities, crystal structure and oxide-ion diffusion pathways of the solid solution composition Ba 7 Nb 3.9 Mo 1.1 O 20.05 . Ba 7 Nb 3.9 Mo 1.1 O 20.05 is found to exhibit a bulk conductivity of 5.8 × 10 −4 S cm −1 at 310 °C, which is higher than those of the “best” oxide-ion conductors. The present work also demonstrates the two-dimensional (2D) oxide-ion O1–O5 diffusion through the interstitial octahedral O5 and lattice tetrahedral O1 sites at a high temperature of 800 °C. Preparation and characterization of Ba 7 Nb 4 MoO 20 -based oxides In this work, we studied the electrical and structural properties of Ba 7 Nb 4 MoO 20 -based materials, because (1) the chemical species in Ba 7 Nb 4 MoO 20 are the same as those in the oxide-ion conductor Ba 3 MoNbO 8.5– δ , (2) Ba 7 Nb 4 MoO 20 has the hexagonal perovskite related structure similar to Ba 3 MoNbO 8.5– δ [28] , [29] , [38] , (3) the crystal structure of Ba 7 Nb 4 MoO 20 contains possible oxide-ion conducting Ba–oxygen (c′) layers as does the structure of Ba 3 MoNbO 8.5- δ , and (4) the bond-valence-based energy barrier for oxide-ion migration of Ba 7 Nb 4 MoO 20 (0.21 eV) is lower than that of Ba 3 MoNbO 8.5– δ (0.51–0.35 eV, See the details in Supplementary Note 1 ). Ba 7 Nb 3.95 Mo 1.05 O 20.025 and Ba 7 Nb 3.9 Mo 1.1 O 20.05 were successfully prepared by solid-state reactions. X-ray powder diffraction (XRD) measurements indicated that Ba 7 Nb 3.95 Mo 1.05 O 20.025 and Ba 7 Nb 3.9 Mo 1.1 O 20.05 have the hexagonal perovskite related structure with trigonal \(P\bar 3m1\) space group (Supplementary Fig. 1 ). Arrhenius plots of bulk conductivities ( σ b ) of Ba 7 Nb 4 MoO 20 [40] , Ba 7 Nb 3.95 Mo 1.05 O 20.025 , and Ba 7 Nb 3.9 Mo 1.1 O 20.05 in dry air are shown in Supplementary Fig. 2 . The σ b of Ba 7 Nb 3.9 Mo 1.1 O 20.05 is the highest among the three compositions. Thus, we focus on the Ba 7 Nb 3.9 Mo 1.1 O 20.05 composition for further detailed studies. The cation atomic ratio of Ba: Nb: Mo = 7.11(14): 3.81(3): 1.126(14) for Ba 7 Nb 3.9 Mo 1.1 O 20.05 determined through X-ray fluorescence (XRF) analyses agreed with that of the nominal composition where the number in parentheses is the standard deviation in the last digit. X-ray photoelectron spectroscopy (XPS) data for the Ba 7 Nb 3.9 Mo 1.1 O 20.05 composition indicated that the valences of Ba, Nb and Mo at room temperature (RT) were +2, +5 and +6, respectively (Ba 2+ 7 Nb 5+ 3.9 Mo 6+ 1.1 O 2– 20.05 ; Supplementary Fig. 3 ). Thermogravimetric measurements of Ba 7 Nb 3.9 Mo 1.1 O 20.05 in dry air between 400 and 900 °C indicate very little weight loss and oxygen deficiency δ in Ba 7 Nb 3.9 Mo 1.1 O 20.05− δ at high temperatures (Supplementary Fig. 4 ). 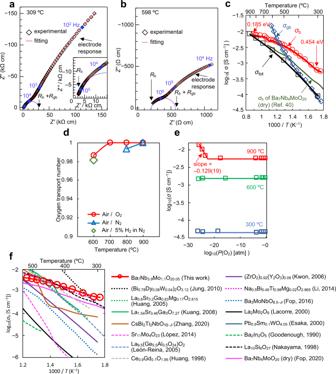Fig. 1: High oxide-ion conductivity of Ba7Nb3.9Mo1.1O20.05. a,bComplex impedance plots of Ba7Nb3.9Mo1.1O20.05recorded in dry air at (a) 309 °C and (b) 598 °C.cArrhenius plots of bulk conductivityσb, grain-boundary conductivityσgband DCσtotof Ba7Nb3.9Mo1.1O20.05in dry air. Activation energy forσbof Ba7Nb3.9Mo1.1O20.05decreases with temperature from 0.454 to 0.185 eV as shown by the red numbers in panel c. Green line representsσbof Ba7Nb4MoO20reported by Fop et al.40.dOxygen transport number of Ba7Nb3.9Mo1.1O20.05.eOxygen partial pressureP(O2) dependence ofσtotof Ba7Nb3.9Mo1.1O20.05.fComparison of bulk conductivities of Ba7Nb3.9Mo1.1O20.05and other oxide-ion conductors. Oxide-ion conduction in Ba 7 Nb 3.9 Mo 1.1 O 20.05 Figure 1a, b shows the typical impedance spectra of Ba 7 Nb 3.9 Mo 1.1 O 20.05 , which indicates the bulk, grain boundary and electrode responses. Bulk conductivity ( σ b ), grain-boundary conductivity ( σ gb ), and grain-boundary capacitance were obtained by the equivalent circuit fitting (Red lines in Fig. 1a, b , Supplementary Figures 5 – 9 ). The σ b and σ gb were measured in dry O 2 , dry air and in dry N 2 at 295 and 598 °C. They were independent of oxygen partial pressure at these temperatures, which indicates ionic conduction (Supplementary Figure 10 ). Figure 1c shows the temperature dependencies of the σ b and σ gb of Ba 7 Nb 3.9 Mo 1.1 O 20.05 on cooling in dry air. The activation energy for σ b was found to be lower than those for σ gb and the DC total electrical conductivity, σ tot . The σ b was higher than σ gb at temperatures below 550 °C and higher than σ tot at temperatures below 850 °C. The oxide-ion transport number ( t ion ) was investigated using oxygen concentration cell measurements. The t ion values were 1.00 between 700 and 900 °C and 0.99 at 600 °C in air/O 2 , 0.99 at 800 °C and 1.00 at 900 °C in air/N 2 , and 0.98 at 600 °C in air/5% H 2 in N 2 (Fig. 1d ). Oxide-ion diffusion in dense Ba 7 Nb 3.9 Mo 1.1 O 20.05 was clearly confirmed by the isotope exchange depth profile method [41] , which calculated a high oxygen tracer diffusion coefficient D * value of 5.35 × 10 –9 cm 2 s –1 at 700 °C and 7.25 × 10 –9 cm 2 s –1 at 800 °C (Supplementary Figure 11 ). The diffusion lengths were about 150 μm and the grain sizes of the Ba 7 Nb 3.9 Mo 1.1 O 20.05 samples were 1–5 μm (Supplementary Figure 12 ), thus, the 18 O tracer species encountered a number of grains and grain boundaries. The total DC electrical conductivity ( σ tot ) was independent of the oxygen partial pressure P (O 2 ) between P (O 2 ) = 7 × 10 −25 ~ 1 atm at 300 °C, P (O 2 ) = 2 × 10 −26 ~ 1 atm at 600 °C, and P (O 2 ) = 5 × 10 −18 ~ 1 atm at 900 °C (Fig. 1e ). Electronic conductivity was observed in the P (O 2 ) range of 6 × 10 −24 ~ 4 × 10 −26 atm at 900 °C with the slope of −0.129(19). Therefore, Ba 7 Nb 3.9 Mo 1.1 O 20.05 exhibits a wider electrolyte domain compared with Ba 7 Nb 4 MoO 20 as reported by Fop et al. [40] . To examine the possible proton conduction of this phase, the DC electrical conductivities, σ tot , of Ba 7 Nb 3.9 Mo 1.1 O 20.05 were measured in wet air (H 2 O partial pressure, P (H 2 O) = 2.3 × 10 −2 atm) and in dry air ( P (H 2 O) < 1.8 × 10 −4 atm). The contribution of protons to σ tot of Ba 7 Nb 3.9 Mo 1.1 O 20.05 was small, even in wet air where the proton transport number was 0.03 − 0.12 (Supplementary Fig. 13 ). Water incorporation behavior was also investigated and the results are shown in Supplementary Fig. 14 and Supplementary Note 2 . A significant but small amount of water uptake was observed for Ba 7 Nb 3.9 Mo 1.1 O 20.05 compared with Ba 7 Nb 4 MoO 20 , which is responsible for the lower transport number of protons in Ba 7 Nb 3.9 Mo 1.1 O 20.05 . These results indicate that the oxide ion is the dominant charge carrier and that Ba 7 Nb 3.9 Mo 1.1 O 20.05 is an oxide-ion conductor. No change was observed in the X-ray powder diffraction patterns before and after the oxygen concentration cell measurements (Supplementary Fig. 15 ), which demonstrates the high phase stability of Ba 7 Nb 3.9 Mo 1.1 O 20.05 at high temperatures and in the wide P (O 2 ) region between P (O 2 ) = 1.2 × 10 −27 and 1 atm. The σ b of Ba 7 Nb 3.9 Mo 1.1 O 20.05 was found to be higher than those of Ba 7 Nb 4 MoO 20 [40] (Fig. 1c ) and YSZ, and comparable to those of the best oxide-ion conductors (Fig. 1f ). It should be noted that the σ b of Ba 7 Nb 3.9 Mo 1.1 O 20.05 was higher than the best oxide-ion conductors at temperatures of around 300 °C, due to the low activation energy of Ba 7 Nb 3.9 Mo 1.1 O 20.05 (0.185-0.454 eV as shown in Fig. 1c ). These results indicate the high potential of the hexagonal perovskite related oxide Ba 7 Nb 3.9 Mo 1.1 O 20.05 as a superior oxide-ion conductor. Fig. 1: High oxide-ion conductivity of Ba 7 Nb 3.9 Mo 1.1 O 20.05 . a , b Complex impedance plots of Ba 7 Nb 3.9 Mo 1.1 O 20.05 recorded in dry air at ( a ) 309 °C and ( b ) 598 °C. c Arrhenius plots of bulk conductivity σ b , grain-boundary conductivity σ gb and DC σ tot of Ba 7 Nb 3.9 Mo 1.1 O 20.05 in dry air. Activation energy for σ b of Ba 7 Nb 3.9 Mo 1.1 O 20.05 decreases with temperature from 0.454 to 0.185 eV as shown by the red numbers in panel c. Green line represents σ b of Ba 7 Nb 4 MoO 20 reported by Fop et al. [40] . d Oxygen transport number of Ba 7 Nb 3.9 Mo 1.1 O 20.05 . e Oxygen partial pressure P (O 2 ) dependence of σ tot of Ba 7 Nb 3.9 Mo 1.1 O 20.05 . f Comparison of bulk conductivities of Ba 7 Nb 3.9 Mo 1.1 O 20.05 and other oxide-ion conductors. Full size image Structural origin of the high oxide-ion conductivity in Ba 7 Nb 3.9 Mo 1.1 O 20.05 Next, we discuss the structural origin of the high oxide-ion conductivity of Ba 7 Nb 3.9 Mo 1.1 O 20.05 , based on its refined crystal structure and neutron scattering length density (NSLD) at 800 °C (Fig. 2 ). In the Rietveld refinements of the neutron-diffraction data, the Mo 6+ and Nb 5+ cations were assumed to be disordered, since they have quite similar neutron scattering lengths. By the trigonal \(P\bar 3m1\) hexagonal perovskite polytype 7H (c′hhcchh; Fig. 2a ), the crystal structure of Ba 7 Nb 3.9 Mo 1.1 O 20.05 was successfully refined by Rietveld analyses of the neutron-diffraction data measured in situ at a temperature of 800 °C in vacuum on the super-high-resolution diffractometer, SuperHRPD [42] , [43] at J-PARC, Japan (Fig. 3 and Supplementary Table 1 ). In order to examine the oxide-ion diffusion pathway and to validate the crystal structure of Ba 7 Nb 3.9 Mo 1.1 O 20.05 , the NSLD was analysed using the maximum-entropy method (MEM) and structure factors obtained through the Rietveld analysis. It is well known that the MEM is a powerful tool to study the structural disorder and ion-diffusion pathways in various ionic conductors [16] , [19] , [31] . Oxygen atoms were found to partially occupy the octahedral interstitial O5 site in the Ba1(O1) 2− x (O5) 0.05+ x layer (Fig. 2a ), because (i) the Rietveld fit for the structural model with the O5 atom (weighted profile reliability factor R wp = 2.39%) was lower than those without the O5 atom ( R wp = 2.47%) and (ii) the MEM NSLD distribution clearly shows the O5 site (Fig. 2b, d ). Here the x in Ba1(O1) 2− x (O5) 0.05+ x is the vacancy content at the O1 site in the unit cell. We applied the split-atom model for the tetrahedral O1 site, because the atomic displacement parameter was quite high for the non-split-atom model and the Rietveld fit for the split-atom model ( R wp = 2.39%) was better than that for the non-split atom model ( R wp = 2.44%). Fig. 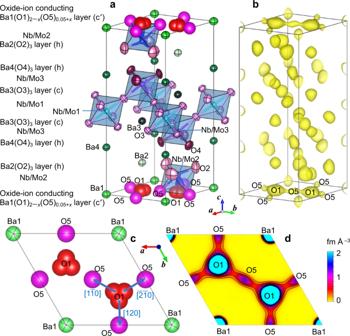Fig. 2: Experimental evidence of the interstitial oxygen O5 and the O1−O5 oxide-ion interstitialcy diffusion of Ba7Nb3.9Mo1.1O20.05at a high temperature of 800 °C. aRefined crystal structure andbcorresponding yellow isosurface of maximum-entropy method neutron scattering length densities (MEM NSLDs) at 0.36 fm Å−3of Ba7Nb3.9Mo1.1O20.05at 800 °C. Refined crystal structure (c) and corresponding MEM NSLD distribution (d) on theabplane atz= 0 of Ba7Nb3.9Mo1.1O20.05at 800 °C. Ind, the contour lines from 0 to 2 fm Å−3by the step of 0.2 fm Å−3. Thermal ellipsoids in panels (a) and (c) are drawn at the 90% probability level. Arrows incdenote the directions of oxide-ion O1-to-O5 migration. 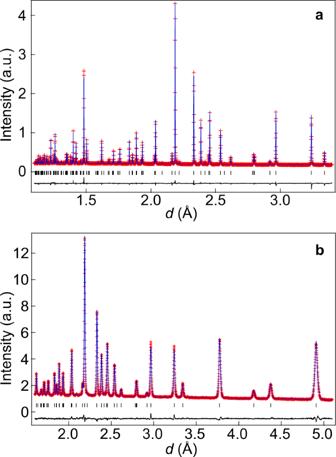Fig. 3: Rietveld patterns of Ba7Nb3.9Mo1.1O20.05at 800 °C. Rietveld patterns of neutron-diffraction data taken with the (a) backscattering bank (d= 1.1−3.4 Å) and (b) 90obank (d= 1.6−5.1 Å) of the SuperHRPD diffractometer in vacuum at 800 °C. The observed and calculated intensities and difference plots are shown by red marks, blue and black solid lines, respectively. Black tick marks stand for calculated Bragg peak positions. 2: Experimental evidence of the interstitial oxygen O5 and the O1−O5 oxide-ion interstitialcy diffusion of Ba 7 Nb 3.9 Mo 1.1 O 20.05 at a high temperature of 800 °C. a Refined crystal structure and b corresponding yellow isosurface of maximum-entropy method neutron scattering length densities (MEM NSLDs) at 0.36 fm Å −3 of Ba 7 Nb 3.9 Mo 1.1 O 20.05 at 800 °C. Refined crystal structure ( c ) and corresponding MEM NSLD distribution ( d ) on the ab plane at z = 0 of Ba 7 Nb 3.9 Mo 1.1 O 20.05 at 800 °C. In d , the contour lines from 0 to 2 fm Å −3 by the step of 0.2 fm Å −3 . Thermal ellipsoids in panels ( a ) and ( c ) are drawn at the 90% probability level. Arrows in c denote the directions of oxide-ion O1-to-O5 migration. Full size image Fig. 3: Rietveld patterns of Ba 7 Nb 3.9 Mo 1.1 O 20.05 at 800 °C. Rietveld patterns of neutron-diffraction data taken with the ( a ) backscattering bank ( d = 1.1−3.4 Å) and ( b ) 90 o bank ( d = 1.6−5.1 Å) of the SuperHRPD diffractometer in vacuum at 800 °C. The observed and calculated intensities and difference plots are shown by red marks, blue and black solid lines, respectively. Black tick marks stand for calculated Bragg peak positions. Full size image The crystal structure of Ba 7 Nb 3.9 Mo 1.1 O 20.05 consists of an oxide-ion conducting Ba1(O1) 2− x (O5) 0.05+ x layer (c′), two Ba2(O2) 3 layers (h), two Ba4(O4) 3 layers (h), two Ba3(O3) 3 layers (c), and Nb and Mo cations at the Nb/Mo1, Nb/Mo2 and Nb/Mo3 sites (Fig. 2a ). A striking feature of the MEM NSLD distribution of Ba 7 Nb 3.9 Mo 1.1 O 20.05 at 800 °C is the connected oxide-ion diffusional pathway between the tetrahedral O1 and interstitial octahedral O5 sites on the oxide-ion conducting Ba1(O1) 2− x (O5) 0.05+ x layer (c′) (Fig. 2b, d ). The oxide ions two-dimensionally migrate through both lattice O1 and interstitial O5 sites, which indicates the interstitialcy mechanism of oxide-ion diffusion. The bond-valence-based energy barriers for oxide-ion migration, E b , for the refined crystal structure of Ba 7 Nb 3.9 Mo 1.1 O 20.05 at 800 °C also supported this 2D feature, because the E b along the ab plane (0.19 eV) is much lower than E b along the c axis (1.54 eV). Ba 7 Nb 3.9 Mo 1.1 O 20.05 has an excess oxygen of x = 0.05 (O 20+ x or O 0.05 in Ba 7 Nb 3.9 Mo 1.1 O 20.05 ) compared with the mother material Ba 7 Nb 4 MoO 20 , which leads to a larger amount of interstitial oxygen and the higher oxide-ion conductivity of Ba 7 Nb 3.9 Mo 1.1 O 20.05 (Fig. 1c ). In conclusion, we have discovered a structure family of rare-earth-free oxide-ion conductors based on the hexagonal perovskite related oxide Ba 7 Nb 4 MoO 20 . Ba 7 Nb 3.9 Mo 1.1 O 20.05 shows a wide stability range and predominantly oxide-ion conduction in the oxygen partial pressure range from 2 × 10 –26 to 1 atm at 600 °C. The bulk conductivity of Ba 7 Nb 3.9 Mo 1.1 O 20.05 is as high as 5.8 × 10 −4 S cm −1 at 310 °C. This high conductivity is ascribed to the interstitial O5 oxygen, 2D oxide-ion O1 − O5 diffusion through the lattice tetrahedral O1 and interstitial O5 octahedral oxygen sites on the ab plane at z = 0 and to the low activation energy for oxide-ion conductivity. The (tetrahedral O1)–(octahedral O5) diffusion pathways in Ba 7 Nb 3.9 Mo 1.1 O 20.05 are along the [ \(1\bar 10\) ], [120] and [ \(\bar 2\bar 10\) ] directions (Arrows in Fig. 2c ), which are the same as those for the (tetrahedral O3)–(octahedral O2) migration paths in the hexagonal perovskite related oxide Ba 3 MoNbO 8.5– δ [31] . This strongly suggests that the (tetrahedral)–(octahedral) oxide-ion migration pathway along the [ \(1\bar 10\) ], [120] and [ \(\bar 2\bar 10\) ] directions on the oxygen deficient c′ layer is a common feature of the oxide-ion conductors with hexagonal perovskite related structures. This feature would be a guide for design of oxide-ion conductors with the hexagonal perovskite-related structures. The present finding of high oxide-ion conductivities in rare-earth-free Ba 7 Nb 3.9 Mo 1.1 O 20.05 suggests the ability of various hexagonal perovskite related oxides as superior oxide-ion conductors. Synthesis and characterization Ba 7 Nb 3.95 Mo 1.05 O 20.025 and Ba 7 Nb 3.9 Mo 1.1 O 20.05 were prepared by the solid-state reactions. High-purity (> 99.9%) BaCO 3 , Nb 2 O 5 , and MoO 3 were mixed and ground using an agate mortar and pestle as ethanol slurries and dry powders repeatedly for 0.5–2 h. The obtained mixtures were calcined at 900 °C for 10–12 h in static air. The calcined samples were crushed and ground using an agate mortar and pestle as ethanol slurries and dry powders repeatedly for 0.5–2 h. The powders thus obtained were uniaxially pressed into pellets at 62–150 MPa and subsequently sintered in static air at 1100 °C for 24 h. Parts of the sintered pellets were crushed and ground into white powders to measure X-ray powder diffraction, atomic absorption spectroscopy (AAS, Hitachi Z-2300), inductively coupled plasma optical emission spectroscopy (ICP-OES, Hitachi PS3520UVDD), and thermogravimetric (TG) data. To identify the existing phases, X-ray powder diffraction patterns of Ba 7 Nb 3.95 Mo 1.05 O 20.025 and Ba 7 Nb 3.9 Mo 1.1 O 20.05 were measured at RT with an X-ray powder diffractometer (BRUKER D8 Advance, Cu K α radiation, 2 θ range: 5−90°). The chemical composition of Ba 7 Nb 3.9 Mo 1.1 O 20.05 was examined by energy dispersive XRF analyses (Rigaku, NEX DE). XPS spectra of Ba 7 Nb 3.9 Mo 1.1 O 20.05 were measured using an X-ray photoelectron spectrometer (ULVAC PHI 5000 Versa Probe III). TG analysis was carried out in dry air using a Bruker-AXS 2020SA instrument at the heating and cooling rates of 10 °C min −1 . The heating and cooling cycle was repeated three times to negate the influence of absorbed species, such as water and to confirm the reproducibility of the measurement. Measurements of electrical conductivity, oxygen diffusion coefficient and transport properties The electrical conductivities of Ba 7 Nb 3.9 Mo 1.1 O 20.05 were measured as a function of temperature by AC impedance spectroscopy in flowing dry air, N 2 , and O 2 gases (100 mL min −1 ) using a sintered pellet (20 mm in diameter, 2.7 mm in thickness, relative density of 100−98%) with Pt electrodes. Impedance spectra were recorded with a Solartron 1260 impedance analyser in the frequency range of 10 MHz−1 Hz at an applied alternating voltage of 100 mV. The activation energies, E a , for the conductivities were estimated using the Arrhenius equation: 
    σ = A_0/Texp(  - E_a/kT)
 (1) where A 0 , k , and T are the pre-exponential factor, Boltzmann constant, and absolute temperature, respectively. Oxygen concentration cell measurements were conducted to investigate the oxygen transport number t ion using a sintered pellet (20 mm in diameter, 4.5 mm in height, and relative density of 100−98%) attached to an alumina tube with a glass seal. One side of the pellet was exposed to flowing dry air and the other side to flowing dry O 2 (Air/O 2 ), N 2 (Air/N 2 ), or 5% H 2 in N 2 (Air/5% H 2 in N 2 ) gases at high temperatures. The electromotive forces of the concentration cell were recorded with a Keithley model 617 electrometer. The following Nernst equation was utilized to estimate the t ion : 
    E = t_ionRT/4Fln( p( O_2)/p^0( O_2))
 (2) where F is the Faraday constant, R is the gas constant, T is the absolute temperature, p (O 2 ) is the oxygen partial pressure of the gas of O 2 , N 2 , 5% H 2 in N 2 , and p 0 (O 2 ) (= 0.21 atm) is the oxygen partial pressure of dry air. After the oxygen concentration cell measurements, the surface of the pellet was ground with sandpaper carefully to remove the Pt paste and then crushed and ground into powder. X-ray diffraction patterns of the resulting powders were measured to investigate the phase stability at high temperatures and different atmospheres. The total electrical conductivity σ tot of the Ba 7 Nb 3.9 Mo 1.1 O 20.05 pellet (relative density: 95%) was measured by a DC-4-probe method with Pt electrodes at various oxygen partial pressure p (O 2 ). The p (O 2 ) was controlled using a mixture of O 2 , N 2 , and 5% H 2 in N 2 and p (O 2 ) was monitored by an oxygen sensor. 18 O tracer diffusion measurements of dense Ba 7 Nb 3.9 Mo 1.1 O 20.05 pellets (relative density of 98-100%) were carried out using the line scan method by secondary ion mass spectrometry (SIMS) [41] . Each sample prepared was polished with diamond spray media down to a finish of 0.25 µm. Samples were pre-annealed in dry research grade oxygen (BOC 99.996%) of natural isotopic abundance for a duration of 10 times that of the isotopic exchange. The samples were subsequently annealed for 2 h in 18 O-enriched gas at a pressure of ≃ 200 mbar. After the exchange anneal, the samples were cut perpendicular to the original surface and the exposed cross-sections polished to 0.25 μm finish, as above. The oxygen diffusion profiles were measured by Time-of-Flight Secondary Ion Mass Spectrometry (ToF-SIMS) using a ToF-SIMS.5 instrument (IONTOF GmbH) using Bi + ions at 25 keV energy. Values of oxygen self-diffusion, D *, and surface exchange, k , coefficients were obtained by fitting the experimental data to Crank’s solution of Fick’s 2 nd law of diffusion [41] , [44] using the TraceX software [45] . The microstructure of the Ba 7 Nb 3.9 Mo 1.1 O 20.05 pellet used for the 18 O tracer diffusion measurements was observed by a scanning electron microscope (KEYENCE VE-8800). Neutron-diffraction measurements of Ba 7 Nb 3.9 Mo 1.1 O 20.05 at 800 °C, Rietveld and MEM analyses High-temperature neutron-diffraction measurements of Ba 7 Nb 3.9 Mo 1.1 O 20.05 pellets (8.7 mm in diameter, 43 mm in height) in a Ti-Zr alloy holder were carried out in vacuum using a super-high-resolution time-of-flight (TOF) neutron diffractometer (SuperHRPD) installed at the Materials and Life Science Experimental Facility of J-PARC, Japan [42] , [43] . The absorption correction was performed using the method given by Rouse and Cooper [46] . The diffraction data were analysed by the Rietveld method using the Z-Rietveld program [47] . The neutron scattering length density distribution was investigated using the MEM. The MEM analysis was carried out with computer program, Dysnomia [48] , using the structure factors obtained in the Rietveld refinement of the neutron diffraction data at 800 °C. The MEM calculations were performed with the unit cell divided into 60 × 60 × 168 pixels. Computation of the bond-valence-based energy barrier for oxide-ion migration The bond-valence-based energy landscapes for a test oxide ion were calculated using the SoftBV [49] software with a spatial resolution of 0.1 Å. The refined crystal structure, MEM neutron scattering length density distributions, and bond-valence-based energy landscape were depicted using VESTA [50] .